Trinuclear zinc complexes for biologically relevant μ3-oxoanion binding and carbon dioxide fixation Tremendous efforts have been made to model multinuclear zinc enzymes. Despite such efforts, it remains a challenge to design single molecules that stabilize μ 3 -oxoanion-bridged trinuclear zinc cores as analogues of enzymatic active sites. The conversion of carbon dioxide to carbonates is a biological process mediated by carbonic anhydrases and a natural process for large-scale carbon dioxide fixation. Here we report a trinuclear zinc scaffold for capturing biologically relevant μ 3 -oxoanions, such as phosphate and carbonate, and its ability to catalytically convert carbon dioxide to carbonates. Structurally characterized {Zn 3 (μ 3 -PO 4 )} and {Zn 3 (μ 3 -CO 3 )} cores are observed in solution by nuclear magnetic resonance and high-resolution mass spectrometry. The activity of the μ 3 -carbonate unit can be sterically controlled, which makes the carbon dioxide fixation cycle feasible. Our results suggest that this trinuclear zinc scaffold catalytically converts carbon dioxide to carbonates under mild conditions and provides a good model for studying oxoanion-bridged zinc cores in solution. Zinc is the second most common metallic element in biological systems and the only one known to be essential for functions of enzymes in all six of the fundamental classes [1] , [2] , [3] . The zinc cation has key roles in enzymatic activity, structural organization and functional regulation due to its strong Lewis acidity and other unusual chemical properties, including rapid ligand exchange, flexible coordination and lack of redox chemistry under physiological conditions [4] . However, the physical properties of Zn(II) make most spectroscopic techniques and methodologies employed for probing other biological metals inapplicable to the characterization of zinc enzymes [2] , [4] . Synthetic zinc models have attracted much attention [5] , [6] , [7] , [8] , [9] , [10] , [11] because they are more amenable to structural, spectroscopic and mechanistic studies that could provide information regarding zinc chemistry and its coordination environment [12] , [13] . Numerous synthetic model complexes have been documented with an emphasis placed on the cleavage of bonds in amides (peptidases and amidases) and in phosphate esters (nucleases, phospholipases, phosphatases and kinases), as well as on the reversible hydration of carbon dioxide (carbonic anhydrases) [5] , [6] , [7] , [8] , [9] , [10] , [11] . Despite these achievements and the discovery that multiple zinc ions in a single molecule endow unique activity [14] , [15] , [16] , [17] , [18] , [19] , synthetic analogues that contain structurally characterized μ 3 -oxoanion (that is, phosphate)-bridged trinuclear zinc cores (to model enzymatic active sites) have yet to be developed. The conversion of CO 2 to carbonate is an important biological process catalysed by carbonic anhydrases that transports CO 2 out of tissues, maintains the acid-base balance and provides a biosynthetic carbon source [4] , [5] , [7] , [13] . Many synthetic efforts have been focused on mimicking this class of zinc enzymes [5] , [7] , [8] , [13] , [20] . However, the condensation between different zinc species complicates the solution study of Zn-bound carbonate and renders the isolation of the zinc bicarbonate complex, which is a critical intermediate in catalysis, very challenging [8] , [20] . CO 2 is a major anthropogenic greenhouse gas, and its continuous accumulation in the atmosphere is thought to be detrimental to the environment, contributing to global warming and climate change [21] , [22] . Therefore, the capture, storage and conversion of CO 2 are important areas of research [22] , [23] , [24] , [25] , [26] , [27] , [28] , [29] , [30] . In nature, large-scale capture and storage are achieved by conversion of CO 2 to carbonates [31] . Valuable inorganic carbonate materials including limestone and soda have been produced and used for millennia. For example, crushed rock, which is primarily composed of calcium carbonate, has been used as building materials, aggregates and chemical feedstocks. In addition, synthetic or precipitated calcium carbonate has primarily been used in the paper, plastics, rubber and paint industries [31] . In addition to the abovementioned aspects, the chemical fixation and activation of CO 2 via transition metal complexes have drawn extensive interest due to the intriguing coordination chemistry of CO 2 (refs 32 , 33 , 34 ) and its hydration products [28] , [35] , [36] , [37] , [38] , [39] . In the zinc area, triply bridging carbonate units are often found in the solid structures of multinuclear zinc complexes and coordination polymers. Although self-assembled trinuclear μ 3 -carbonate species that have adequate stability in solution are known for other metal systems [39] , those based on zinc are intrinsically less stable and thus more difficult to analytically intercept in solution [8] , [28] , [36] , [40] , [41] . To gain more insight into the coordination dynamics of carbonate and zinc, especially those with triply bridging carbonate units, it is necessary to develop μ 3 -carbonate trinuclear zinc species that have sufficient and controllable stability and that are amenable to solution studies. Herein, we report a trinuclear zinc scaffold and its ability to capture biologically relevant μ 3 -oxoanions and catalytically convert CO 2 to carbonates. The trinucleating ligand N(CH 2 - o -C 6 H 4 -CH 2 N(CH 2 py) 2 ) 3 ( L , py=pyridine), which was recently reported by Lippard and co-workers [42] , [43] by appending three dipicolylamine (DPA) units to a tris(xylyl)amine scaffold, is used to synthesize complex [Zn 3 L (CF 3 SO 3 ) 6 ] ( 1 ), μ 3 -phosphate complex [Zn 3 (CF 3 SO 3 ) 3 (μ 3 -HPO 4 ) L ](CF 3 SO 3 ) ( 2 ) and the μ 3 -carbonate complex [Zn 3 (CF 3 SO 3 ) 3 (μ 3 -CO 3 ) L ](CF 3 SO 3 ) ( 3 ) ( Fig. 1 ). Complex 2 is the first example of a synthetic {Zn 3 (μ 3 -PO 4 )} core stabilized in a single ligand framework that mimics the natural zinc core of enzymes [42] such as P1 nuclease [44] , [45] and phospholipase C [46] , [47] . The stability in solution of the μ 3 -oxoanions is evaluated via multinuclear nuclear magnetic resonance (NMR) and high-resolution mass spectrometry (HRMS). The activity of the μ 3 -carbonate can be sterically controlled using the complex [Zn 3 (OH 2 ) 3 (μ 3 -CO 3 ) L ](ClO 4 ) 4 ( 4 ). These features are crucial for catalytic CO 2 fixation to carbonates and for studying the solution behaviour of oxoanion-bridged zinc species. 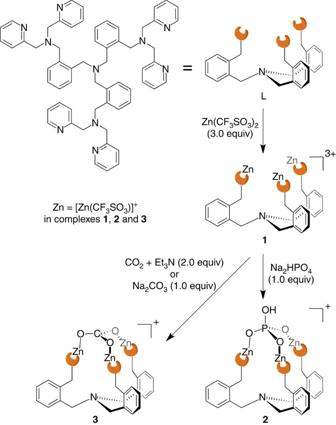Figure 1: Schematic representation of ligand L and synthesis of complexes 1–3. Trinucleating ligandLhas three DPA units attached to the ortho positions of a tris(xylyl)amine scaffold. The zinc-based tripodal scaffold1is able to capture a phosphate or a carbonate ion to produce the trinuclear zinc complexes2and3with μ3-HPO4and μ3-CO3, respectively. The carbonate in3can also be generated upon CO2fixation using1. Figure 1: Schematic representation of ligand L and synthesis of complexes 1–3. Trinucleating ligand L has three DPA units attached to the ortho positions of a tris(xylyl)amine scaffold. The zinc-based tripodal scaffold 1 is able to capture a phosphate or a carbonate ion to produce the trinuclear zinc complexes 2 and 3 with μ 3 -HPO 4 and μ 3 -CO 3 , respectively. The carbonate in 3 can also be generated upon CO 2 fixation using 1 . Full size image Syntheses and characterization of complexes 2 and 3 Biomimetic complexes for trinuclear zinc enzymes are rare [9] . Our interest in studying zinc coordination and catalysis led us to generate trinuclear zinc complexes that are able to bind μ 3 -oxoanions of biological significance (for example, phosphate and carbonate) [4] , [8] , [9] , [13] . Tris-DPA ligand L , which contains a tris(xylyl)amine scaffold and three DPA coordination moieties [42] , [43] , was chosen. The tris(xylyl)amine scaffold provides the appropriate symmetry and spacing to model trinuclear zinc enzymes [42] , and DPA is widely used as a Zn(II) chelator with good binding affinity [48] . The reaction of L and three equivalents of Zn(CF 3 SO 3 ) 2 in an inert atmosphere yielded complex 1 ( Fig. 1 and Supplementary Fig. S1 , see Methods and Supplementary Methods for details). Subsequent treatment of 1 with an equimolar sample of Na 2 HPO 4 yielded complex 2 . X-ray diffraction studies revealed that 2 crystallized in trigonal space group R 3c (the crystal data and structure refinement details are summarized in Supplementary Table S1 ). The monocationic cluster of 2 is located at a special position with a crystallographically required C 3 axis passing through the central phosphate (P1 and O1) and nitrogen (N1) atoms ( Fig. 2a ). The three symmetric, DPA-appended ligand arms of L each coordinate one Zn(II) ion through three nitrogen atoms, and the phosphate group triply bridges these Zn(II) ions through three facial oxygen atoms. The distorted trigonal–bipyramidal coordination sphere of each Zn ion is saturated by a triflate ligand with one sulphonate oxygen (O3, Zn1−O3, 2.129(5) Å) and the tertiary nitrogen atom (N2, Zn1−N2, 2.264(5) Å) of DPA at two apexes. For the phosphate group, its P1−O1 bond distance of 1.576(8) Å is much longer than that of P1−O2, which is 1.507(4) Å, indicating that this fourth uncoordinated oxygen atom (that is, O1) is protonated [42] . The one additional CF 3 SO 3 − counterion per trimetallic cluster was also located in the X-ray structure. 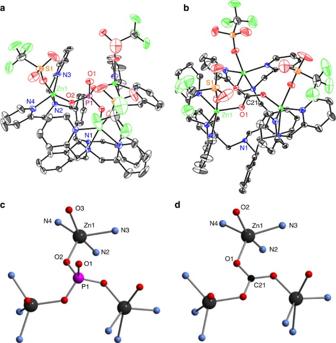Figure 2: Solid-state structures of 2 and 3. (aandb), Thermal ellipsoid plots (50% probability) of the X-ray structures of the monocationic clusters of2and3, respectively. The hydrogen atoms are omitted for clarity. TheC3axis passes through the O1, P1 and N1 atoms inaand through the C21 and N1 atoms inb. (candd), Ball-and-stick representations of the truncated {Zn3(μ3-PO4)} and {Zn3(μ3-CO3)} cores in2and3, respectively. Selected bond lengths in Å: (c), Zn1–O2 1.914(4), Zn1–O3 2.129(5), Zn1–N2 2.264(5), Zn1–N3 2.047(5), Zn1–N4 2.051(5), P1–O1 1.576(8) and P1–O2 1.507(4). (d) Zn1–O1 1.937(4), Zn1–O2 2.146(5), Zn1–N2 2.281(5), Zn1–N3 2.031(5), Zn1–N4 2.063(5) and C21–O1 1.278(4). Figure 2: Solid-state structures of 2 and 3. ( a and b ), Thermal ellipsoid plots (50% probability) of the X-ray structures of the monocationic clusters of 2 and 3 , respectively. The hydrogen atoms are omitted for clarity. The C 3 axis passes through the O1, P1 and N1 atoms in a and through the C21 and N1 atoms in b . ( c and d ), Ball-and-stick representations of the truncated {Zn 3 (μ 3 -PO 4 )} and {Zn 3 (μ 3 -CO 3 )} cores in 2 and 3 , respectively. Selected bond lengths in Å: ( c ), Zn1–O2 1.914(4), Zn1–O3 2.129(5), Zn1–N2 2.264(5), Zn1–N3 2.047(5), Zn1–N4 2.051(5), P1–O1 1.576(8) and P1–O2 1.507(4). ( d ) Zn1–O1 1.937(4), Zn1–O2 2.146(5), Zn1–N2 2.281(5), Zn1–N3 2.031(5), Zn1–N4 2.063(5) and C21–O1 1.278(4). Full size image Complex 2 was directly detected in solution by multinuclear NMR and HRMS studies. One singlet at 1.79 p.p.m. was observed in the 31 P NMR ( Supplementary Fig. S2 ). A strong peak at 1655.1074 was observed for monocation [Zn 3 (CF 3 SO 3 ) 3 (μ 3 -HPO 4 ) L ] + in the positive mode mass spectrum ( m / z ), which matches the calculated value of 1655.1050 for [C 63 H 61 F 9 N 10 O 13 PS 3 Zn 3 ] + ( Supplementary Fig. S3 ). In the 13 C NMR spectrum, all 11 aromatic and 3 aliphatic carbon signals of the ligand backbone were successfully located ( Fig. 3b ). The 13 C− 19 F coupling in the triflate ions caused the CF 3 carbon peak to be split with a ratio of 1:3:3:1 and the two stronger peaks were observed in the spectrum. These results demonstrate that the molecular structure of 2 remains intact in solution. 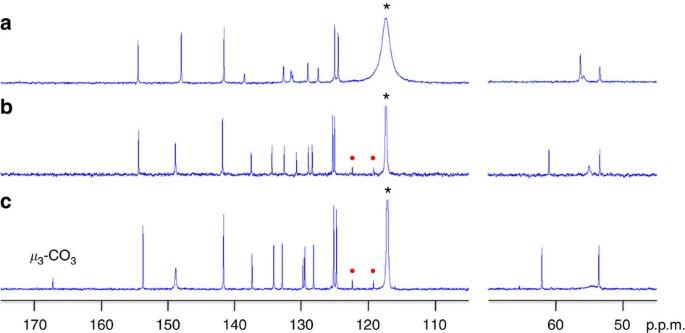Figure 3:13C NMR spectra of trinuclear zinc complexes. (a)13C NMR of [Zn3L(CF3SO3)6] (1). (b)13C NMR of [Zn3(CF3SO3)3(μ3-HPO4)L](CF3SO3) (2). (c)13C NMR of [Zn3(CF3SO3)3(μ3-CO3)L](CF3SO3) (3). The13C signal of the CF3SO3−anion inbandcis split into a quartet with a ratio of 1:3:3:1, and the two stronger peaks are indicated (·). The μ3-CO3unit in3is observed by13C NMR spectroscopy, which shows a strong singlet at 167.1 p.p.m.. All spectra were obtained in acetonitrile-d3(solvent signals were marked using *). Figure 3: 13 C NMR spectra of trinuclear zinc complexes. ( a ) 13 C NMR of [Zn 3 L (CF 3 SO 3 ) 6 ] ( 1 ). ( b ) 13 C NMR of [Zn 3 (CF 3 SO 3 ) 3 (μ 3 -HPO 4 ) L ](CF 3 SO 3 ) ( 2 ). ( c ) 13 C NMR of [Zn 3 (CF 3 SO 3 ) 3 (μ 3 -CO 3 ) L ](CF 3 SO 3 ) ( 3 ). The 13 C signal of the CF 3 SO 3 − anion in b and c is split into a quartet with a ratio of 1:3:3:1, and the two stronger peaks are indicated (·). The μ 3 -CO 3 unit in 3 is observed by 13 C NMR spectroscopy, which shows a strong singlet at 167.1 p.p.m.. All spectra were obtained in acetonitrile-d 3 (solvent signals were marked using *). Full size image Because the triply bridging CO 3 2− and PO 3 (OH) 2− ions have the same C 3 symmetry and anionic charges, and the sizes of their trigonal plane defined by three coordinating oxygen atoms are comparable, we replaced Na 2 HPO 4 with Na 2 CO 3 in the reaction with 1 . The resultant sample behaved very similar to 2 in proton NMR studies, which indicate that 1 is also able to capture a carbonate anion to form a {Zn 3 (μ 3 -CO 3 )} cluster. To further examine its potential for CO 2 fixation, we exposed a freshly prepared methanol solution of 1 to CO 2 in the presence of two equivalents of triethylamine. The resultant clear solution was stirred for 1 h followed by drying in vacuo to yield an off-white solid. The slow vapour diffusion of diethyl ether to an acetonitrile solution of this solid afforded complex 3 as colourless cubes (yield 85%). In carbonic anhydrases, a Zn(II)-bound hydroxo group nucleophilically attacks one CO 2 molecule to generate a bicarbonate ion [8] , [13] . The same reaction could occur in our system, except that the resultant bicarbonate ion is trapped in the trinuclear zinc cavity via rapid condensation with a neighbouring {Zn(II)−OH} unit (vide infra) [8] . In carbonic anhydrases, the bicarbonate ion readily releases due to its low binding affinity in the enzymatic active site [13] . As we expected, the X-ray structure of 3 is similar to that of 2 , in which a {Zn 3 (μ 3 -CO 3 )} core is coordinated by ligand L with each Zn(II) ion bound to three nitrogen atoms of one DPA-appended ligand arm ( Fig. 2b ). The monocationic cluster of 3 has the crystallographically required C 3 axis passing through atom C21 of the central μ 3 -carbonate and atom N1. Each Zn(II) ion has a fifth triflate ligand to produce a distorted trigonal–bipyramidal coordination geometry. In comparison to 2 , the trimetallic cluster of 3 is slightly squeezed, and the Zn···Zn separation of 4.896 Å in 3 is shorter than that of 5.271 Å in 2 ( Fig. 2c ). We rationalized that this structural change is due to the fact that the trigonal plane defined by the three coordinating oxygen atoms of CO 3 2− in 3 has an O···O separation of 2.214 Å, whereas the separation is 2.489 Å for HPO 4 2− in 2 ( Fig. 2c ). The three symmetric C21−O1 bond distances of 1.278(4) Å and O1−C21−O1 bond angles of 119.96(5)° are consistent with a μ 3 -carbonate ion. Analysis of the infrared spectra of 2 and 3 defined the carbonate-related vibration in 3 at 1,473 cm −1 , which is consistent with the reported range for symmetrically bridging μ 3 -carbonate groups [32] . Remarkably, this carbonate was observed with 13 C NMR spectroscopy as a sharp singlet at 167.1 p.p.m. ( Fig. 3c ), and all of the other signals from the tripodal ligand backbone and triflate anions in both 2 and 3 are in good agreement. These results indicate that the molecular structure of 3 remains intact in solution. In addition, the monocationic unit of 3 was also detected in the HRMS studies (Found: 1619.1261; calcd. for [C 64 H 60 F 9 N 10 O 12 S 3 Zn 3 ] + =1619.1285, Supplementary Fig. S4 ). The activity of 3 in solution The conversion of CO 2 to carbonate is one of the key steps in catalytic CO 2 fixation. In carbonic anhydrases, the facile release of the bicarbonate ligand from Zn(II) is a crucial requirement for their activity [8] . To examine the potential for such Zn-based tripodal species to serve as artificial carbonic anhydrases, we determined whether the μ 3 -carbonate unit could be removed from 3 . The binding constant of a carbonate anion in the trinuclear zinc cavity of 1 was determined to be 1.23 × 10 5 M −1 ( Supplementary Figs. S5 and S6 ). This result suggests that the μ 3 -carbonate in 3 could be extracted using calcium ions due to the small solubility product constant of CaCO 3 (2.80 × 10 −9 ) [49] . A similar strategy was previously used by Bouwman and co-workers to regenerate a dinuclear copper complex for electrocatalytic CO 2 fixation in which the Cu(II)-bound oxalate ligands were precipitated as lithium oxalate from acetonitrile [29] . However, attempts to remove the carbonate unit by mixing 3 and calcium triflate in acetonitrile were unsuccessful. No precipitate was observed, even when a large excess (10 equivalents) of calcium ions was added either at room temperature or under elevated temperatures up to 80 °C. The structural analysis of the X-ray structure of 3 revealed that its {Zn 3 (μ 3 -CO 3 )} core was sterically protected by both the tripodal ligand framework of L and the three Zn-bound triflate groups. As shown in the space-filling diagrams of the monocationic cluster of 3 ( Fig. 4a and b ), the μ 3 -carbonate unit is entirely encapsulated in the ligand backbone, which may prevent the carbonate ion from interacting with the calcium ions in solution. Therefore, the {Zn 3 (μ 3 -CO 3 )} core of 3 remains unaffected in the presence of calcium under the above conditions. To remove the μ 3 -carbonate unit and complete the catalytic cycle as we have proposed for CO 2 fixation ( Fig. 5a ), it is necessary to tune the steric property around the {Zn 3 (μ 3 -CO 3 )} core. One method is to use small and/or non-coordinating anions to replace the bulky triflate groups. As shown in Fig. 4c and d , by removing the three Zn-bound triflate ligands, the {Zn 3 (μ 3 -CO 3 )} core to a large extent is exposed to the exterior environment, and the central carbonate ion in such a structural conformation is believed to be accessible by other reagents. 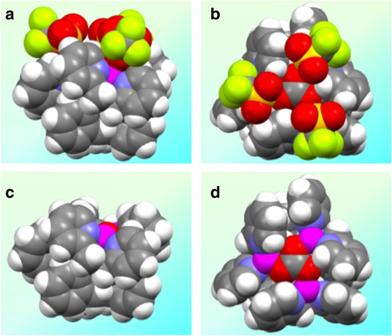Figure 4: Space-filling diagrams of the X-ray structure of 3. (aandb) Side view and top view of the monocationic cluster of3, showing that the μ3-CO3unit is sterically protected by the tripodal ligand framework ofLand the three Zn-bound triflate groups. (candd) Side view and top view of the monocationic cluster of3without the three Zn-bound triflate ligands, indicating that the μ3-CO3unit is now accessible by external calcium ions. Figure 4: Space-filling diagrams of the X-ray structure of 3. ( a and b ) Side view and top view of the monocationic cluster of 3 , showing that the μ 3 -CO 3 unit is sterically protected by the tripodal ligand framework of L and the three Zn-bound triflate groups. ( c and d ) Side view and top view of the monocationic cluster of 3 without the three Zn-bound triflate ligands, indicating that the μ 3 -CO 3 unit is now accessible by external calcium ions. 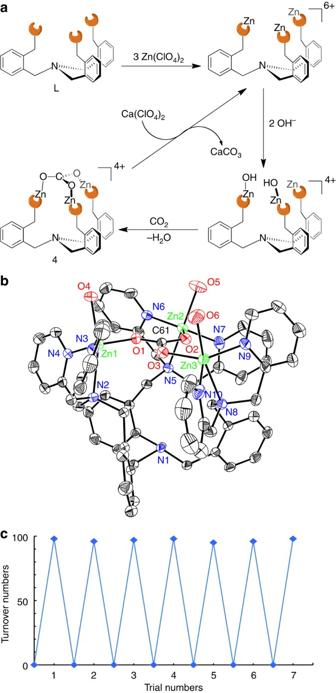Figure 5: Schematic of CO2fixation in the presence of tripodal Zn complex. (a) Proposed catalytic cycle for CO2fixation on a trinuclear Zn core. (b) Thermal ellipsoid plot (50% probability) of intermediate4. The hydrogen atoms are omitted for clarity. (c) Catalytic conversion of CO2to carbonates using [Zn3L](ClO4)6. After each run, the catalyst was recovered and reused in the next trial, and a nearly constant catalytic activity for the fixation of CO2was observed. Full size image Figure 5: Schematic of CO 2 fixation in the presence of tripodal Zn complex. ( a ) Proposed catalytic cycle for CO 2 fixation on a trinuclear Zn core. ( b ) Thermal ellipsoid plot (50% probability) of intermediate 4 . The hydrogen atoms are omitted for clarity. ( c ) Catalytic conversion of CO 2 to carbonates using [Zn 3 L ](ClO 4 ) 6 . After each run, the catalyst was recovered and reused in the next trial, and a nearly constant catalytic activity for the fixation of CO 2 was observed. Full size image Synthesis and structure of complex 4 Because of the steric effect, we synthesized the perchlorate analogue of 3 by reacting ligand L with Zn(ClO 4 ) 2 . Exposure of this reaction mixture to CO 2 and subsequent crystallization from acetonitrile yielded complex 4 as colourless prisms (yield 81%). Crystallographic studies revealed that 4 crystallized in triclinic space group P ( Supplementary Table S1 ). The structure of 4 resembles that of 3 , except that the three Zn-bound triflate ions in 3 are replaced by three aqua ligands in 4 ( Fig. 5b ). All three Zn(II) ions have a distorted trigonal–bipyramidal coordination with typical Zn(II)−N bond distances (2.024(3)−2.058(3) Å for equatorial; 2.253(3)−2.306(3) Å for axial) and Zn(II)−O bond lengths (1.927(2)−1.937(2) Å for μ 3 -CO 3 2− oxygen; 2.084(3)−2.106(3) Å for aqua oxygen). The central carbonate unit has an average C−O bond length of 1.281(4) Å, which is a value that is nearly identical to that found in 3 . Four perchlorate anions were also located in the X-ray structure. In the 13 C NMR spectrum, the carbonate unit of 4 exhibited a sharp singlet at 166.9 p.p.m. ( Supplementary Fig. S7 ). In the HRMS, monocation [Zn 3 (ClO 4 ) 3 (μ 3 -CO 3 ) L ] + was also observed (calcd. for [C 61 H 60 N 10 O 15 Cl 3 Zn 3 ] + =1469.1174, found: 1469.1260, Supplementary Fig. S8 ). These results confirmed the solution structure of 4 and indicated that the μ 3 -carbonate trinuclear zinc cluster was stable in ligand L even in the absence of the three protecting triflate groups. Catalytic CO 2 transformation studies The solution stability of 4 allows for subsequent activity studies. In contrast to 3 , the addition of an equimolar sample of calcium perchlorate in water to an acetonitrile solution of 4 at room temperature resulted in the immediate precipitation of CaCO 3 with a quantitative yield. The resultant trinuclear zinc complex [Zn 3 L (ClO 4 ) 6 ] ( 5 ) was also characterized ( Supplementary Methods ). The disappearance of the carbonate singlet at 166.9 p.p.m. in the 13 C NMR ( Supplementary Fig. S7 ) and the detection of monocation [Zn 3 L (ClO 4 ) 5 ] + in the HRMS (calcd. for [C 60 H 60 N 10 Cl 5 O 20 Zn 3 ] + =1607.0297, found: 1607.0289, Supplementary Fig. S8 ) were all consistent with the removal of a μ 3 -carbonate unit from 4 . As we proposed in Fig. 5a , this step is essential for the completion of the CO 2 fixation cycle. After establishing the catalytic cycle, we subsequently performed the catalytic conversion of CO 2 to calcium carbonate to evaluate the potential for such trinuclear zinc complexes to serve as artificial carbonic anhydrases. Bubbling CO 2 into a solution containing the [Zn 3 L (ClO 4 ) 6 ] catalyst (0.0032, mmol) and 100 equivalents of calcium perchlorate resulted in the rapid precipitation of CaCO 3 , and ~ 100 turnovers were obtained in a half hour (the reaction rate was limited by the slow addition of triethylamine as the base). The calcium carbonate precipitate was collected by filtration, and its weight (30.5 mg, 0.31 mmol, yield 96%) corresponded to a nearly quantitative conversion of CO 2 to the desired carbonates. More significantly, the proton NMR spectrum of the catalyst recovered from this reaction was the same as that of 4 ( Supplementary Fig. S9 ), which indicated that after the consumption of calcium, the trinuclear zinc species reacted further with CO 2 to generate the μ 3 -carbonate complex 4 . In addition, the recovered catalyst was able to perform this chemistry with nearly identical efficiencies when subjected to new trials of CO 2 fixation under the same conditions. This process could be repeated multiple times, and the catalyst exhibited unchanged activities in all of the runs ( Fig. 5c shows seven repeating cycles). All of the results presented above clearly show the importance of these trinuclear zinc complexes for modelling zinc enzymes [9] , as well as the feasibility of precisely controlling the activity of carbonate-bridged zinc complexes by tuning the zinc coordination. In carbonic anhydrases, the bicarbonate anion generated by the nucleophilic attack of an active zinc hydroxide derivative to CO 2 can be readily displaced with water to complete the catalytic cycle [9] . In contrast, in biomimetic studies, the zinc centre is not adequately protected as it is in nature. Therefore, the condensation between {Zn(II)−OH} and {Zn(II)−OCO 2 H} typically yields multinuclear bridging carbonate species [8] , which makes the isolation of terminal zinc bicarbonate complexes corresponding to the {Zn(II)−OCO 2 H} intermediate in catalysis extremely challenging (the first structurally characterized such species was reported only recently [20] ). The solution stability of carbonate-bridged multinuclear zinc complexes is dependent on the coordination modes of their carbonate ligands. For carbonate-bridged trinuclear zinc complexes, the typical monodentate coordination of the μ 3 -carbonate to each Zn(II) centre is sensitive to hydrolysis [8] , [28] , [36] , [40] , [41] . To better understand the coordination dynamics and the activity of Zn(II)-bound carbonate, it is valuable to first stabilize carbonate-bridged zinc units using well-designed ligand systems and then investigate their solution behaviours. Therefore, we synthesized μ 3 -carbonate trinuclear zinc complexes using trinucleating ligand L . Our results demonstrate that the {Zn 3 (μ 3 -CO 3 )} core encapsulated in L has sufficient stability in solution due primarily to the appropriate symmetry and spacing and the bulky ligand environment produced by L . Importantly, the activity of the μ 3 -carbonate in our system can be sterically controlled. The {Zn 3 (μ 3 -CO 3 )} core in 4 is much more susceptible to calcium than that in 3 because 3 gains additional protection from coordinating triflate groups. It is necessary to note that our studies show that ligand L has a vital role in catalytic CO 2 fixation. A comparison of the association constant of Zn(II) and DPA (1.43 × 10 7 M −1 ) [48] and the solubility product constant of zinc carbonate (1.46 × 10 −10 ) [49] indicates that mononuclear [Zn(DPA)] [2] + species are not stable in the presence of carbonate ions. Control experiments confirmed that the addition of sodium carbonate to a solution of [Zn(DPA)](ClO 4 ) 2 resulted in the immediate precipitation of ZnCO 3 . In contrast to mononuclear species, trinuclear zinc complexes 3 and 4 retained their structures in solution even with a large excess of carbonate ions (10 equivalents, Supplementary Fig. S5 ). These results suggest that 3 and 4 are resistant to the demetalation of zinc under catalytic conditions. In addition, based on our observations, a triply bridging carbonate unit is involved in the catalysis with these trinuclear zinc complexes. First, the condensation between {Zn(II)−OH} and {Zn(II)−OCO 2 H} is extremely rapid in solution [8] . For example, it has been previously demonstrated [8] that the use of sterically demanding tris(pyrazolyl)borato (TP RR′ ) ligands is necessary for stabilizing zinc bicarbonate species because the reduced steric demands of the Pr i versus Bu t substituents of the TP RR′ ligands cause the immediate formation of a dinuclear bridging carbonate complex in the reaction between {Zn(II)−OH} and CO 2 . Because the intramolecular reaction between neighbouring {Zn(II)−OCO 2 H} and {Zn(II)−OH} in ligand L should be much easier and the steric effect of the DPA group for each zinc centre is small, their condensation to yield bridging carbonate species will be straightforward. Second, control experiments using mononuclear [Zn(DPA)](ClO 4 ) 2 as the catalyst resulted in the demetalation of zinc from DPA and deactivation of the catalyst. Third, complex [Zn 3 L (CF 3 SO 3 ) 6 ] ( 1 ) is nearly ineffective in catalysing the conversion of CO 2 to calcium carbonate. We rationalize that the rapid condensation between {Zn(II)−OH} and {Zn(II)−OCO 2 H} gives the μ 3 -carbonate trinuclear zinc complex 3 , which does not further react with calcium ion and inhibits the catalytic cycle. The combination of these results suggests that the formation of a triply bridging carbonate unit in the trinuclear zinc cores is faster than the formation of calcium carbonate, and such a bridging carbonate unit is relevant to CO 2 fixation catalysis in our studies. The catalytic CO 2 fixation of this trinuclear zinc system is different from the dinuclear copper complex reported by Bouwman and co-workers [29] , as discussed below. First, the {Zn 3 } system is more efficient than the {Cu 2 } complex in catalytic CO 2 sequestration and conversion to the desired products. Because of the rate-limiting electroreduction of Cu(II) to Cu(I), only six turnovers were obtained during 7 h of catalysis using the {Cu 2 } complex. In addition, the precipitation of the generated lithium oxalate onto the electrode surface hampers electron transfer, which further decreases the catalytic efficiency of the {Cu 2 } complex. Second, the {Zn 3 } system catalyses the conversion of CO 2 to calcium carbonate under mild conditions, whereas in the {Cu 2 } system, electrical energy is required to reduce Cu(II) to the active Cu(I) species to complete the catalytic cycle. Third, the formation of the μ 3 -carbonate intermediate in the {Zn 3 } system is an intramolecular process, but an intermolecular reaction occurs to produce the μ 2 -oxalate bridged tetranuclear Cu(II) complex. This difference may be critical in diluted systems because the dimerization rate depends on the second-order concentration of the {Cu 2 } species. To improve the catalytic efficiency, immobilization of {Cu 2 } complex onto the electrode surface was proposed. However, the dimerization of immobilized {Cu 2 } species may be challenging. Fourth, although the dinuclear Cu(I) complex was oxidized by CO 2 rather than O 2 in air, interference from other redox active molecules has not been excluded. For example, it was reported that the {Cu 2 } complex can be oxidized by chloroform [29] . For the {Zn 3 } system, the catalyst is redox inert and robust during CO 2 fixation. In conclusion, trinuclear zinc scaffold 1 is used to capture biologically relevant oxoanions. The μ 3 -phosphate complex 2 is the first structurally characterized synthetic analogue containing a {Zn 3 (μ 3 -PO 4 )} core in a single ligand framework mimicking natural zinc enzyme cores. The μ 3 -carbonate complexes 3 and 4 are generated by CO 2 fixation. All three complexes are directly observed in solution by NMR and HRMS techniques, and the activity of the triply bridging carbonate can be sterically controlled to provide good models for studying bridging carbonates. This trinuclear zinc scaffold can catalyse the conversion of CO 2 to carbonates under mild conditions with the involvement of a triply bridging carbonate unit. General considerations Manipulations of air- and moisture-sensitive materials were performed under an atmosphere of nitrogen gas using standard Schlenk line techniques. Ligand L is synthesized according to the reported procedure [42] with modifications to improve both yields and purities. All of the other reagents were purchased from commercial suppliers and used as received unless otherwise noted. All newly synthesized complexes were characterized by 1 H, 13 C and 31 P (for 2 ) NMR spectroscopy, FTIR (for 2 , 3 and 4 ), high-resolution ESI-MS, single-crystal X-ray diffraction (for 2 , 3 , and 4 ) and confirmed by elemental analysis for purity. High-resolution mass spectra of final ligand L and trinuclear zinc complexes 1–5 in acetonitrile were acquired on a Brüker Fourier Transform Ion Cyclotron Resonance Mass Spectrometer APEX IV at Peking University. For experimental details and complete characterization of all new complexes, see Supplementary Methods . Synthesis of complex 1 To a stirred solution of ligand L (30 mg, 0.032 mmol) in 10 ml dichloromethane at room temperature, three equivalents of Zn(CF 3 SO 3 ) 2 (36 mg, 0.097 mmol) dissolved in methanol (2 ml) were added. The resultant clear solution was stirred under nitrogen until the solvent was completely evaporated at room temperature. Then, the residue was carefully washed with diethyl ether and dried in vacuo to yield a light-yellow sticky solid (58 mg, yield 90%). Synthesis of complex 2 To a stirred solution of ligand L (30 mg, 0.032 mmol) in 10 ml dichloromethane at room temperature, Zn(CF 3 SO 3 ) 2 (36 mg, 0.097 mmol) dissolved in methanol (2 ml) was added. The resultant clear solution was stirred for 1 h under nitrogen followed by dropwise addition of Na 2 HPO 4 (4.6 mg, 0.032 mmol) in H 2 O (1 ml). When the solvent was completely dried in vacuo at room temperature, the residue was extracted using acetonitrile. Slow vapour diffusion of diethyl ether into this acetonitrile solution at room temperature yielded colourless prisms of complex 2 in three days (53 mg, yield 90.2%). Synthesis of complex 3 To a stirred solution of ligand L (30 mg, 0.032 mmol) in 10 ml dichloromethane at room temperature, Zn(CF 3 SO 3 ) 2 (36 mg, 0.097 mmol) dissolved in methanol (2 ml) was added, followed by 9 μl of triethylamine (0.065 mmol). The resultant clear solution was stirred for 1 h under an atmosphere of carbon dioxide, and then, the solvent was completely dried in vacuo at room temperature. Next, the residue was extracted using acetonitrile. Slow vapour diffusion of diethyl ether into this acetonitrile solution at room temperature yielded colourless prisms of complex 3 in three days (50 mg, yield 85.2%). Synthesis of complex 4 The procedure for synthesizing 4 is similar to that for 3 except that Zn(ClO 4 ) 2 ·6H 2 O (36 mg, 0.097 mmol) was used and crystals of 4 were obtained at −20 °C in 3 weeks (43 mg, yield 81.2%). Carbonate removal studies of 4 To a stirred solution of 4 (32 mg, 0.020 mmol) in 10 ml acetonitrile at room temperature, Ca(ClO 4 ) 2 (5.3 mg, 0.022 mmol) dissolved in water (2 ml) was added. The resultant mixture was stirred for 1 h under nitrogen followed by centrifugation to yield a pellet of CaCO 3 (1.8 mg, yield 90%). The clear supernatant was concentrated in vacuo, and the residue was carefully washed with diethyl ether to give a light-yellow sticky solid of complex [Zn 3 L (ClO 4 ) 6 ] ( 5 ) (27 mg, yield 80%). Catalysis studies To a stirred solution of ligand L (3.0 mg, 0.0032, mmol) in 10 ml methanol at room temperature, Zn(ClO 4 ) 2 ·6 H 2 O (3.6 mg, 0.0097, mmol) was added. After stirring this solution under nitrogen for 1 h, 2 ml of aqueous solution of Ca(ClO 4 ) 2 (76.8 mg, 0.32 mmol) was added. Then, the resultant solution was stirred for 30 min under an atmosphere of carbon dioxide, during which time 90 μl of triethylamine (0.65 mmol) was constantly being added to this solution using a syringe pump. The precipitate that formed was collected by centrifugation, washed with water ( × 3) and methanol ( × 3) and dried in vacuo to produce a pellet of CaCO 3 (30.5 mg, yield 95%). The filtrate was dried in vacuo followed by extraction with water. The residue collected by centrifugation was dried and subjected to a new trial of catalysis studies. Control experiments using the same conditions without [Zn 3 L (ClO 4 ) 6 ], with [Zn(DPA)](ClO 4 ) 2 (4.6 mg, 0.01 mmol) or with [Zn 3 L (CF 3 SO 3 ) 6 ] (6.5 mg, 0.0032, mmol) were also performed, which yielded <1.0 mg of CaCO 3 (yield <3%). X-ray diffraction studies Complete data sets for 2 , 3 , and 4 were collected. Single crystals suitable for X-ray analysis were each coated with Paratone-N oil, suspended in a small fibre loop and placed in a cooled gas stream on a Brüker APEX CCD X-ray diffractometer. The diffraction intensities were measured using graphite monochromated Mo K α radiation ( λ =0.71073 Å) at 173(2) or 153(2) K. Data collection, indexing, data reduction and final unit cell refinements were performed using APEX2 (ref. 50 ), and absorption corrections were applied using the SADABS program [51] . All of the structures were solved with direct methods using SHELXS [52] and refined against F 2 on all of the data by full-matrix least squares with SHELXL [53] following established refinement strategies [54] . Details are provided in the Supplementary Methods and Supplementary Data 1–3 . Thermal ellipsoid plots of complexes 2–4 are shown in Supplementary Figs. S10, S11, and S12 , respectively. Accession codes: The X-ray crystallographic coordinates for structures reported in this article have been deposited at the Cambridge Crystallographic Data Centre (CCDC), under deposition number CCDC 931955 (complex 2 ), 931956 (complex 3 ), and 931957 (complex 4 ). These data can be obtained free of charge from The Cambridge Crystallographic Data Centre via www.ccdc.cam.ac.uk/data_request/cif . How to cite this article: Liu, X. et al. Trinuclear zinc complexes for biologically relevant μ 3 -oxoanion binding and carbon dioxide fixation. Nat. Commun. 4:2375 doi: 10.1038/ncomms3375 (2013).